Shoot-derived cytokinins systemically regulate root nodulation Legumes establish symbiotic associations with nitrogen-fixing bacteria (rhizobia) in root nodules to obtain nitrogen. Legumes control nodule number through long-distance communication between roots and shoots, maintaining the proper symbiotic balance. Rhizobial infection triggers the production of mobile CLE-RS1/2 peptides in Lotus japonicus roots; the perception of the signal by receptor kinase HAR1 in shoots presumably induces the production of an unidentified shoot-derived inhibitor (SDI) that translocates to roots and blocks further nodule development. Here we show that, CLE-RS1/2-HAR1 signalling activates the production of shoot-derived cytokinins, which have an SDI-like capacity to systemically suppress nodulation. In addition, we show that LjIPT3 is involved in nodulation-related cytokinin production in shoots. The expression of LjIPT3 is activated in an HAR1-dependent manner. We further demonstrate shoot-to-root long-distance transport of cytokinin in L. japonicus seedlings. These findings add essential components to our understanding of how legumes control nodulation to balance nutritional requirements and energy status. To establish symbiotic associations with rhizobia, a group of nitrogen-fixing bacteria, leguminous plants form nodules on their roots in response to rhizobial infection. The rhizobia colonize these nodules, supplying host plants with fixed atmospheric nitrogen while receiving photosyntates in turn. While such a symbiotic relationship generally is beneficial to both partners, the formation of excessive numbers of nodules inhibits the growth of the host plants. To avoid this effect, plants perform autoregulation of nodulation (AON), which systemically controls the number of nodules [1] . AON is a long-distance negative-feedback system involving root–shoot communication [2] , [3] , [4] . In the legume Lotus japonicus , two leucine-rich repeat receptor-like kinases, HYPERNODULATION ABERRANT ROOT FORMATION 1 (HAR1) and KLAVIER, have been identified as key components of AON that function in shoots [5] , [6] , [7] , [8] , [9] . The two proteins are orthologous to Arabidopsis CLAVATA1 and RECEPTOR-LIKE PROTEIN KINASE 2, respectively, which are involved in the maintenance of stem cell populations in shoot apical meristems via short-range cell-to-cell communication [10] , [11] . As an underlying mechanism of AON, it has been postulated that signalling substances are produced in roots upon rhizobial infection, which then are transported to the shoot [2] , [4] . The perception of these primary signals in the shoot generates secondary signals. These shoot-derived signals, also called shoot-derived inhibitors (SDIs), are transported to the roots where they inhibit the initiation of new nodule development [2] , [4] , [12] , [13] , [14] , [15] . In L. japonicus , two peptides, CLE-ROOT SIGNAL 1 (CLE-RS1) and CLE-RS2, are strong candidates for root-derived mobile signalling molecules. Expression of the corresponding genes is induced specifically in infected roots, and CLE-RS2 glycopeptides are transported in the xylem to the shoot where they directly bind to HAR1 (refs 16 , 17 ). Application of arabinosylated CLE-RS peptides to shoots suppresses nodulation in an HAR1-dependent manner [17] . Furthermore, the TOO MUCH LOVE (TML) F-box protein recently has been identified as a root-acting AON factor that inhibits nodulation downstream of HAR1 (refs 18 , 19 ). Although these results provide some insight into signalling mechanisms between the root and shoot, the mechanism and regulation of AON inhibition of nodule development remain mostly unclear. In particular, the identification of the SDI is lacking. In this study, we focused on downstream events of the CLE-RS1/2-HAR1 signalling pathway. We show that the production of cytokinins (CKs) in shoots is activated by rhizobial infection, and that application of exogenous CKs to shoots can inhibit nodulation in a TML-dependent manner. Our results suggest that shoot-derived CKs systemically regulate root nodulation in AON. Phenotypic analyses and quantification of phytohormones The har1 mutant shows a hypernodulation phenotype, possibly because of defects in SDI production [4] , [8] . On the other hand, rhizobial infection induces constitutive expression of CLE-RS1 or RS2 , which encode peptides acting as ligands of HAR1, and inhibits further nodulation, probably due to increased SDI production in the shoot [4] , [16] , [17] . Consequently, we hypothesized that SDI levels in shoots should differ between the har1 mutant and the CLE-RS1/2 constitutive expression lines. If so, candidate SDIs should be identifiable by comparison of metabolite profiles between the different lines. To this end, we generated stable L. japonicus transgenic plants in which either CLE-RS1 or RS2 were overexpressed under the control of the CaMV 35S promoter ( CLE-RS1/2 ox, Supplementary Fig. 1 ). As controls, plants expressing the GUS gene were generated (MG-20 background). Control plants ( GUS ox), har1-7 mutants, CLE-RS1 ox and RS2 ox plants were inoculated with Mesorhizobium loti , and nodules were counted 2 weeks after inoculation. har1-7 plants formed approximately three times more nodules than the control, whereas CLE-RS1 ox and RS2 ox did not form nodules ( Fig. 1a,d–g ). This result was consistent with previous observations of nodulation inhibition by root-specific CLE-RS1 and RS2 expression following hairy root transformation [16] . In addition, we found that lateral root numbers in CLE-RS1 ox and RS2 ox were decreased to 18% and 27%, respectively, of that in control plants ( Fig. 1b,h,j,k ). On the other hand, har1-7 plants formed approximately twice as many lateral roots as control plants ( Fig. 1b,h,i ). Thus, in terms of nodule and lateral root numbers, the CLE-RS1/2 ox phenotypes were opposite to those of the har1-7 mutant. To see whether the nodulation inhibitory effects of CLE-RS1/2 overexpression are mediated through the shoots, we performed reciprocal grafting of shoots and roots between MG-20 (wild type), har1-7 mutants, CLE-RS1 ox and RS2 ox plants ( Fig. 1c ). Shoots of CLE-RS1 ox and RS2 ox inhibited nodulation in both wild-type and har1-7 mutant rootstocks, indicating that CLE-RS1 and RS2 ox expression in the shoots is sufficient to block nodulation. Furthermore, the inhibition of nodulation in rootstocks overexpressing CLE-RS1/2 was suppressed by shoots of har1-7 mutants. These results confirmed that CLE-RS1/2 inhibited nodulation through shoot–root communication in an HAR1-dependent manner, as observed previously [16] . Likewise, shoots from CLE-RS1 ox plants inhibited lateral root formation in both wild-type and har1-7 mutant rootstocks ( Supplementary Fig. 2 ), suggesting that lateral root formation was inhibited by CLE-RS1 expression in the shoot. 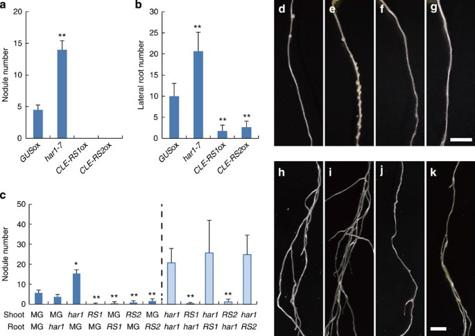Figure 1: Overexpression ofCLE-RS1andRS2inhibit nodulation and lateral root formation. (a) Nodule number inGUSox,har1-7mutant andCLE-RS1/2ox plants (n=6). Nodules were counted 14 days after infection withM. loti. (b) Lateral root numbers (n=6–10) at 21 days after germination in the absence of rhizobia. (c) Shoot-to-root reciprocal grafting between MG-20,har1-7mutant andCLE-RS1/2ox plants (n=6–9). Nodules were counted 14 days after infection. Bars in (a–c) represent means±s.d. Asterisks indicate statistically significant differences from the control (a,b:GUSox,c: MG-20 orhar1-7) at *P<0.05 and **P<0.01, according to the Student’st-test (a,b) and Tukey HSD (c). (d–k) Nodulation phenotypes (d–g) and root phenotypes (h–k) ofGUSox(d,h),har1-7mutant (e,i),CLE-RS1ox (f,j) andRS2ox (g,k). Bars, 5 mm ingford–g, 1 cm inkforh–k. Figure 1: Overexpression of CLE-RS1 and RS2 inhibit nodulation and lateral root formation. ( a ) Nodule number in GUS ox, har1-7 mutant and CLE-RS1/2 ox plants ( n =6). Nodules were counted 14 days after infection with M. loti . ( b ) Lateral root numbers ( n =6–10) at 21 days after germination in the absence of rhizobia. ( c ) Shoot-to-root reciprocal grafting between MG-20, har1-7 mutant and CLE-RS1/2 ox plants ( n =6–9). Nodules were counted 14 days after infection. Bars in ( a – c ) represent means±s.d. Asterisks indicate statistically significant differences from the control ( a , b : GUS ox, c : MG-20 or har1-7 ) at * P <0.05 and ** P <0.01, according to the Student’s t -test ( a , b ) and Tukey HSD ( c ). ( d – k ) Nodulation phenotypes ( d – g ) and root phenotypes ( h – k ) of GUSox ( d , h ), har1-7 mutant ( e , i ), CLE-RS1 ox ( f , j ) and RS2 ox ( g , k ). Bars, 5 mm in g for d – g , 1 cm in k for h – k . Full size image Recently, it was reported that SDI is a small amphiphilic compound (possiblemolecular mass <10 kDa) unlikely to be a protein or an RNA molecule [12] , [13] , [14] , [15] . The har1 mutant shows developmental alterations, including short primary roots and enhanced lateral root formation [5] . In contrast, the numbers of lateral roots were decreased in CLE-RS1 ox and RS2 ox plants ( Fig. 1b ). Therefore, we assumed that SDI might affect plant development in addition to its effects on nodule formation. Plant development is controlled by phytohormones, which are low-molecular mass compounds [15] . Some phytohormones act as long-distance signals in the integrative regulation of development and in defence responses [20] , [21] , [22] . Thus it seemed the obvious next step to compare phytohormone compositions in MG-20 shoots with those of har1-7 mutant and CLE-RS1/2 ox shoots. Given that SDI is produced downstream of CLE-RS1/2 and HAR1 (refs 2 , 16 ), we focused on phytohormones combining two trends, namely increased levels in shoots of both CLE-RS1 ox and CLERS2 ox plants, and decreased levels in har1-7 mutant shoots. In three independent analyses, only one of 39 compounds examined consistently showed both trends, namely iPRPs, which are intermediates of CK biosynthesis ( Table 1 ; Supplementary Table 1 ). In addition, the amount of iPRPs in MG-20 shoots was significantly increased following rhizobial infection, reaching about twice the level detected in non-infected plants ( Fig. 2 ). CKs are transferred from roots to shoots through the xylem [23] , [24] , and tZ-type CKs contribute the largest fraction of translocated CKs [25] . tZ-type CK levels in shoots were unaffected by rhizobial infection ( Fig. 2 ). Thus, increased iPRPs levels in shoots probably are caused by CK synthesis rather than by CKs import from roots. In Arabidopsis , iPRP production is an initial step of CK biosynthesis, and controls the total amount of CKs [26] . Taken together, our results suggested that during nodulation, the production of CKs is induced in shoots through the activation of the CLE-RS1/2-HAR1 signalling pathway. Table 1 Comparison of phytohormone levels between shoots of MG-20, har1-7 mutants and CLE-RS1/2 ox plants. 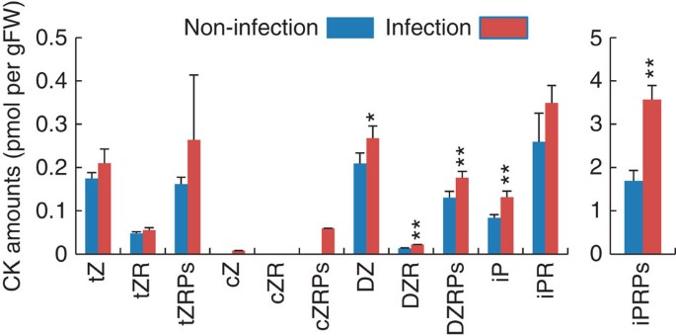Figure 2: iPRPs levels in shoots are increased by rhizobial infection. CK levels in shoots were determined at 5 days after infection withM. loti(infection) or in the absence of rhizobia (non-infection). Means±s.d. from three independent experiments are shown. Asterisks indicate statistically significant differences between treatments (*P<0.05, **P<0.01; Student’st-test). Full size table Figure 2: iPRPs levels in shoots are increased by rhizobial infection. CK levels in shoots were determined at 5 days after infection with M. loti (infection) or in the absence of rhizobia (non-infection). Means±s.d. from three independent experiments are shown. Asterisks indicate statistically significant differences between treatments (* P <0.05, ** P <0.01; Student’s t -test). Full size image CK-feeding assay To investigate whether CKs accumulating in shoots have SDI-like activities, we applied various concentrations of 6-benzylaminopurine (BAP) to MG-20, har1 and tml seedlings via cut surfaces of cotyledons. Application of 10 −6 and 10 −5 M BAP to MG-20 seedlings decreased the number of nodules to 44% and 13%, respectively, compared with the buffer-only control treatment ( Fig. 3a ). Similarly, BAP inhibited nodulation in har1-7 seedlings in a dose-dependent manner ( Fig. 3a ). Evidently, CK applied to shoots inhibits the nodulation through a mechanism downstream of HAR1 action. The inhibitory effect was not observed in plants carrying the tml mutation ( Fig. 3a ), indicating that TML , which functions in roots downstream of HAR1, is required for the inhibitory action of CK. 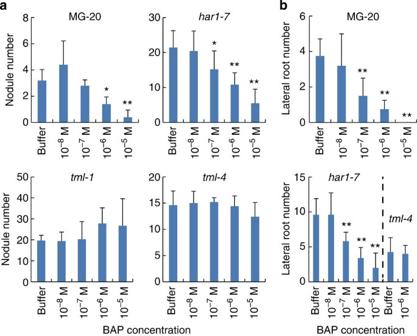Figure 3: BAP suppresses nodulation and lateral root formation in a TML-dependent manner. (a) Effects on nodulation of BAP application to shoots in MG-20 andhar1-7,tml-1andtml-4mutants (n=5). Distal halves of cotyledons were removed at 2 days after germination, and BAP was fed to the cut surfaces. Plants were inoculated withM. loti1 day after starting BAP application. Nodules were counted 14 days after infection. (b) Effects on lateral root formation of BAP application to shoots in MG-20,har1-7andtml-4mutants (n=5). Lateral roots were counted 21 days after starting BAP application in the absence of rhizobia. Data presented are means±s.d. Asterisks indicate statistically significant differences at *P<0.05 and **P<0.01, according to the Student’st-test. Figure 3: BAP suppresses nodulation and lateral root formation in a TML-dependent manner. ( a ) Effects on nodulation of BAP application to shoots in MG-20 and har1-7 , tml-1 and tml-4 mutants ( n =5). Distal halves of cotyledons were removed at 2 days after germination, and BAP was fed to the cut surfaces. Plants were inoculated with M. loti 1 day after starting BAP application. Nodules were counted 14 days after infection. ( b ) Effects on lateral root formation of BAP application to shoots in MG-20, har1-7 and tml-4 mutants ( n =5). Lateral roots were counted 21 days after starting BAP application in the absence of rhizobia. Data presented are means±s.d. Asterisks indicate statistically significant differences at * P <0.05 and ** P <0.01, according to the Student’s t -test. Full size image We further examined effects of CK feeding on lateral root formation, which was affected in CLE-RS1/2 ox, as well as on nodule formation ( Fig. 1b ). The formation of lateral roots was inhibited by BAP fed to shoots; lateral root numbers in MG-20 were decreased to 40% and 20% of the control by 10 −7 and 10 −6 M BAP, respectively ( Fig. 3b ). The application of BAP to the shoot also inhibited lateral root formation in har1-7 mutants ( Fig. 3b ). tml mutants had similar lateral root numbers as MG-20, but the formation rate was not decreased by the BAP treatment ( Fig. 3b ), suggesting that shoot-derived CK controls lateral root formation as well as nodulation in a TML -dependent manner. In Arabidopsis , the phloem has been demonstrated to be capable of transporting large amounts of CKs [27] . We applied labelled CK [28] to establish whether CK fed to leaves is transported to roots in L. japonicus . In fact, the labelled CK soon was detected in root tips ( Table 2 ; Supplementary Table 2 ). Evidently, CKs in the cotyledon are transported to the root tip in L. japonicas ; thus it is likely that exogenously applied BAP ( Fig. 3 ) was transported through the phloem to the root. Table 2 Labelled CK applied to cotyledons is transported to the root tip. Full size table Expression analyses of L. japonicus IPT genes in shoots Quantification of phytohormones had shown that CLE-RS1/2 ox shoots accumulated significantly larger amounts of iPRPs than MG-20 shoots. iPRPs are synthesized at initial steps of the CK biosynthetic pathway in a reaction catalysed by isopentenyltransferase (IPT). These steps are rate limiting in CK production, suggesting that production of iPRPs and CK levels are regulated by the expression of IPTs [26] , [29] . Six IPT genes ( LjIPT ) can be found in the L. japonicus genomic database [30] . We examined the expression patterns of these LjIPT genes of MG-20, har1-7 mutants and CLE-RS1/2 ox plants during nodulation ( Fig. 4a,b ; Supplementary Fig. 3 ). Among the five LjIPT genes for which activity could be detected, LjIPT1 and LjIPT3 showed increased expression in MG-20 shoots starting at 1 and 3 days, respectively, after inoculation. The other three LjIPT genes showed no response ( Supplementary Fig. 3 ). Responses of LjIPT1 and LjIPT3 genes were not observed in har1-7 shoots ( Fig. 4a ; Supplementary Fig. 3 ). Moreover, the expression of LjIPT3 was constitutively increased in CLE-RS1 ox and RS2 ox plants in the absence of rhizobia ( Fig. 4b ). The timing of the induction of LjIPT3 expression was consistent with the timing of the initiation of AON reported previously [31] . These findings suggested that the activation of LjIPT3 in the shoot is closely related to AON activation. 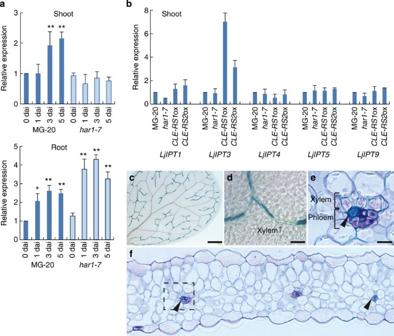Figure 4: Expression analyses ofLjIPTgenes. (a) Relative expression ofLjIPT3genes in shoots and roots of MG-20 andhar1-7plants at different times after infection withM. loti(dai). Dai, days after infection. Asterisks indicate statistically significant differences at *P<0.05 and **P<0.01, according to the Student’st-test. (b) Relative expression ofLjIPTsgenes in shoots of various plant lines grown in the absence of rhizobia. Expression ofLjIPT2was not detected. (a,b) Data presented are means±s.d. of three biological repeats. Transcript amounts in different samples were normalized to those of ubiquitin. (c,d) GUS staining in leaves ofProLjIPT3:GUSplants at 3 days after infection withM. loti. (e,f) Cross-section of a leaf stained with 0.05% toluidine blue. The arrowhead highlights an area showing the GUS signal. (e) Magnified image of the boxed region inf. Bars, 0.5 mm (c), 50 μm (d,f), 10 μm (e). Figure 4: Expression analyses of LjIPT genes. ( a ) Relative expression of LjIPT3 genes in shoots and roots of MG-20 and har1-7 plants at different times after infection with M. loti (dai). Dai, days after infection. Asterisks indicate statistically significant differences at * P <0.05 and ** P <0.01, according to the Student’s t -test. ( b ) Relative expression of LjIPTs genes in shoots of various plant lines grown in the absence of rhizobia. Expression of LjIPT2 was not detected. ( a , b ) Data presented are means±s.d. of three biological repeats. Transcript amounts in different samples were normalized to those of ubiquitin. ( c , d ) GUS staining in leaves of ProLjIPT3:GUS plants at 3 days after infection with M. loti . ( e , f ) Cross-section of a leaf stained with 0.05% toluidine blue. The arrowhead highlights an area showing the GUS signal. ( e ) Magnified image of the boxed region in f . Bars, 0.5 mm ( c ), 50 μm ( d , f ), 10 μm ( e ). Full size image We next examined the expression pattern of LjIPT3 in roots. Expression of LjIPT3 is induced in MG-20 roots by rhizobial infection, as shown recently ( Fig. 4a ) [30] . This infection-dependent activation was also observed in har1-7 ( Fig. 4a ), suggesting that, unlike in the case of shoots, HAR1 is not required for the activation of LjIPT3 in roots. In addition, the timing of LjIPT3 activation differs between shoots and roots; activation was observed 3 days after inoculation in shoots, but as early as 1 day after inoculation in roots ( Fig. 4a ). We examined spatial expression patterns of LjIPT3 in shoots using transgenic ProLjIPT3:GUS plants, in which a 2.0-kb fragment of the LjIPT3 promoter region was inserted upstream of the GUS reporter gene. GUS signals were detected along a subset of leaf veins ( Fig. 4c,d ). Detailed analyses of leaf cross-sections showed the signal restricted to phloem tissue ( Fig. 4e,f ). This pattern resembled that of HAR1 , which had been reported previously [32] . Functional analysis of the LjIPT3 gene To elucidate the function of LjIPT3 in AON, we identified mutant lines with LORE1 retrotransposon inserts in the coding sequence of LjIPT3 ( Supplementary Fig. 4 ) [33] , [34] . In addition, we produced transgenic plants overexpressing LjIPT3 under the control of the CaMV 35S promoter ( LjIPT3 ox; Supplementary Fig. 1 ). In LjIPT3 shoots, iPRPs levels were five times higher than in MG-20 shoots in the absence of rhizobia ( Supplementary Fig. 5 ), suggesting that overexpression of LjIPT3 is sufficient to increase iPRPs levels. LjIPT3 ox lines and Ljipt3 mutants exhibited opposite phenotypes in terms of nodule number. LjIPT3 ox lines formed only 30–40% of the nodule number found in MG-20, whereas nodule numbers in Ljipt3 mutants exceeded those in Gifu B-129 by 58% ( Fig. 5a–e ). Evidently, LjIPT3 expression negatively influences nodulation. Furthermore, reciprocal grafting analysis showed that Ljipt3 shoots increased the number of nodules formed on Gifu B-129 rootstocks, while nodule numbers were comparable between Ljipt3 and Gifu B-129 rootstocks carrying Gifu B-129 shoots ( Fig. 5f ). These results demonstrated that LjIPT3 functions in the shoot-dependent inhibition of nodulation. The negative effect of LjIPT3 expression in the shoot was confirmed by grafting LjIPT3 ox shoots onto MG-20 wild-type rootstocks ( Fig. 5g ). As we also observed a reduction of nodule numbers in LjIPT3 ox rootstocks carrying MG-20 shoots, the expression of LjIPT3 in roots appeared to inhibit nodulation as well ( Fig. 5g ). 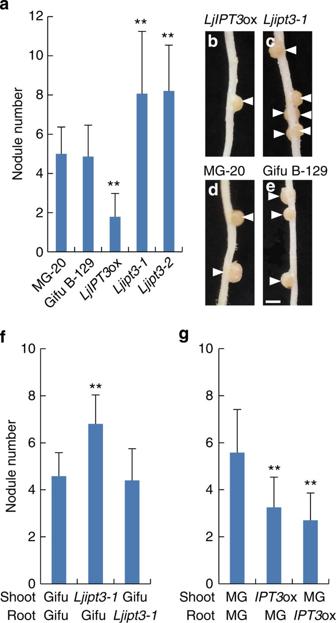Figure 5: LjIPT3 effects on nodule number. (a) Nodule number of wild type (MG-20 and Gifu B-129),LjIPT3ox plants (MG-20 background) andLjipt3mutants (Gifu B-129 background) (n=14–15). (b–e) Nodule phenotypes, arrowheads indicate nodules. (f,g) Nodule numbers in shoot-to-root reciprocal grafts between Gifu B-129 andLjipt3-1mutants (n=10–12) (f) and between MG-20 andLjIPT3ox (n=10–12) (g). Nodules were counted 21 days after infection withM. loti. Data presented are means±s.d. Asterisks indicate statistically significant differences at **P<0.01 according to the Student’st-test. Bar, 1 mm. Figure 5: LjIPT3 effects on nodule number. ( a ) Nodule number of wild type (MG-20 and Gifu B-129), LjIPT3 ox plants (MG-20 background) and Ljipt3 mutants (Gifu B-129 background) ( n =14–15). ( b – e ) Nodule phenotypes, arrowheads indicate nodules. ( f , g ) Nodule numbers in shoot-to-root reciprocal grafts between Gifu B-129 and Ljipt3-1 mutants ( n =10–12) ( f ) and between MG-20 and LjIPT3 ox ( n =10–12) ( g ). Nodules were counted 21 days after infection with M. loti . Data presented are means±s.d. Asterisks indicate statistically significant differences at ** P <0.01 according to the Student’s t -test. Bar, 1 mm. Full size image Site of AON action in the root To identify potential sites of AON action in the root, we examined the interaction between CLE-RS and CK signalling involving LHK1. Proper nodule development requires LHK1 , which encodes a putative CK receptor [35] , [36] . Initially, we performed grafting using rootstocks of hit1 and snf2 mutants, which are loss-of- and gain-of-function mutants of LHK1 , respectively. It seems that the hit1 mutation reduces the number of nodules due to defective CK signalling in roots [35] , while the snf2 mutation causes the formation of so-called spontaneous nodules in the absence of rhizobia [36] . Grafting analysis showed that CLE-RS1 ox shoots inhibited nodulation in hit1-1 and spontaneous nodulation in snf2 rootstocks ( Supplementary Fig. 6 ). These results suggested that the site of AON action in roots may be downstream of LHK1. In Medicago truncatula , CK signalling involving MtCRE1, a counterpart of LHK1, may be involved in nodulation by mediating NSP2 expression [37] . Therefore, we investigated the relationship between NSP2 expression and CLE-RS1/2 overexpression. In CLE-RS1 ox and RS2 ox plants, NSP2 expression was downregulated to 15% and 40%, respectively, of that in control plants (MG-20) ( Supplementary Fig. 7 ). Thus, AON seems to suppress the expression of NSP2 downstream of LHK1. AON systemically regulates the number of root nodules through shoot–root communication [2] , [4] . The inhibition of the formation of excess root nodules by a shoot-derived signal is a key element of AON, but molecular mechanisms involved in the production of the shoot-derived signal are poorly understood. We have shown that CLE-RS1/2-HAR1 signalling activates CK production in shoots, and that the synthesized CKs inhibit nodulation. TML, a component of AON acting in roots, is required for the inhibitory action of CKs. Thus, these results suggest that the inhibition of nodulation caused by CKs is under the control of AON especially between HAR1 and TML ( Fig. 6 ). Our data also indicate that LjIPT3 is involved in CK production during nodulation. LjIPT3 expression is activated in shoots in an HAR1-dependent manner. Genetic analysis indicates that LjIPT3 acts as a negative regulator of nodulation. Since the nodulation phenotype of Ljipt3 knockout mutants is milder than that of canonical AON mutants, several LjIPT genes may function redundantly in the control of nodulation. Generally, Arabidopsis IPT genes seem to have overlapping functions in diverse processes of plant development [38] . Promoter–reporter analyses showed that the LjIPT3 promoter was active specifically in phloem cells, suggesting that CKs may be synthesized in the shoot phloem upon rhizobial infection of roots ( Fig. 6 ). In Arabidopsis , iP-type CKs are transported from shoot to root via phloem sieve tubes [25] , [39] , and we demonstrated that CKs are transported from cotyledons to root tips in L. japonicus . In addition, in our grafting experiments nodulation was inhibited when LjIPT3 ox plants were used as scions ( Fig. 5g ), consistent with the notion that shoot-derived CKs inhibit nodulation in roots. 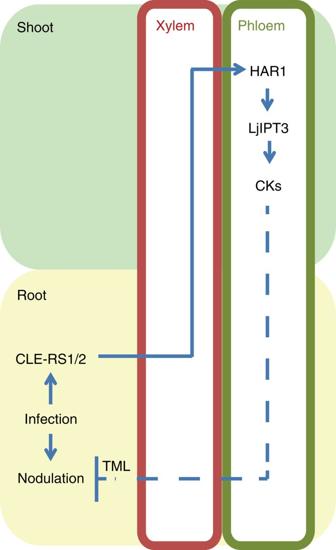Figure 6: Schematic illustration of the proposed AON model. Demonstrated and putative regulatory relationships are indicated by bold and dotted lines, respectively. See text for details. Figure 6: Schematic illustration of the proposed AON model. Demonstrated and putative regulatory relationships are indicated by bold and dotted lines, respectively. See text for details. Full size image CKs have long been suggested to act as positive regulators of nodule development. For example, a nodulation-deficient Rhizobium mutant could be recovered by introducing a gene related to trans -zeatin secretion [40] , and recent genetic analyses demonstrated that activation of CK signalling in host plants is necessary and sufficient to form nodule primordia [35] , [36] , [41] . Moreover, LjIPT3 is involved in CK production in roots with positive effects on nodulation [30] . In contrast, our results showed a negative effect of shoot-derived CKs on nodulation, as CKs act systemically to restrict the number of nodules. The production of CKs in both shoots and roots during nodulation is induced by expression of LjIPT3 , but the timing of LjIPT3 activation is different between shoots and roots. In addition, our data also indicated that LjIPT3 expression in shoots is induced in an HAR1-dependent manner, whereas HAR1 is not required for the activation of LjIPT3 in roots. These findings suggest that CKs, which negatively affect nodulation, may be produced following AON signalling in shoots, whereas CKs with positive effects on nodulation may be produced independently of AON signalling in roots. Therefore, different induction mechanisms including differential timing of CK production and HAR1 dependence can provide CKs with a dual role in nodulation. The visible loss-of-function phenotypes of LjIPT3 might differ drastically between different lines due to the dual role of CKs. RNA interference knockdown lines of LjIPT3 decrease nodule number, probably because the nodulation-promoting function of LjIPT3 is predominantly affected in this case [30] . In contrast, knockout lines used in the present study ( Ljipt3-1 and Ljipt3-2 ) showed increased nodule numbers, presumably because of defects in the nodulation-restricting role of LjIPT3 in shoots. In this case, any inhibition of the positive effects of LjIPT3 in roots does not become apparent. Our grafting experiment and expression analysis suggested that AON may suppress NSP2 expression downstream of LHK1. CK application to roots significantly downregulates NSP2 expression after a transient upregulation [37] . Similarly, shoot-derived CKs may control the number of nodules by downregulating NSP2 expression. Our grafting experiment also showed that AON retains its inhibitory effects on nodulation in the LHK1 mutant background. L. japonicus has three putative CKs receptors with overlapping functions in the control of nodulation [42] . On the basis of these findings and our present results, we hypothesize that CKs with negative effects on nodulation may suppress the expression of NSP2 via CK receptor(s) other than LHK1. Such differential function of CK receptors may explain the dual role of CKs. On the other hand, we cannot rule out the possibility that additional components induced downstream of CK production in shoots act systemically to inhibit nodulation. We showed that CKs produced in shoots block the formation of lateral roots in a TML-dependent manner. This implies that nodulation and lateral root formation are systemically regulated via the same pathway downstream of CK production in the shoot. Although tml-4 mutants were insensitive to shoot-applied CKs with regard to the inhibition of lateral root formation, lateral root numbers of the mutants were similar to that of the wild type. This suggests that the TML regulation of lateral root development depends on additional factors. For instance, nitrate influences both lateral root development and nodulation [43] , [44] , [45] . Nodulation is suppressed by nitrate, and AON factors such as HAR1, KLV and TML are involved in this inhibitory regulation [1] , [2] , [5] , [6] , [18] . Nitrate systemically regulates root architecture, and induces IPT3 expression in Arabidopsis shoots [44] , [46] , [47] . Thus, CKs may play a central role in the systemic regulation of root lateral organ development. However, the underlying mechanisms remain obscure. KISS ME DEADLY, a Kelch repeat F-box protein that resembles TML, acts as a negative regulator of CK signalling in Arabidopsis [19] , [48] . Thus, interactions between CKs and TML may be essential for the negative regulation of nodulation, as well as lateral root development by CKs. Further investigations focusing on the interaction between CKs and TML will elucidate how CKs achieve their dual function in the control of nodule development, and may give insights into the long-distance regulatory mechanism required for nodulation and lateral root development. Plant materials and growth conditions We used L. japonicus accessions Miyakojima MG-20 and Gifu B-129 as the wild type, and the Ljipt3-1 and Lipt3-2 LORE1 retrotransposon insertion lines with plant IDs 30001893 and 30012123, respectively. Hypernodulation mutants used were har1-7 (ref. 18 ), tml-1 and tml-4 (ref. 19 ). Mutants of LHK1 were hit1-1 (ref. 35 ) and snf2 (ref. 9 ). Plants were grown in autoclaved vermiculite supplemented with Broughton and Dilworth (B&D) solution [49] with 0.5 mM KNO 3 under 16 h light/8 h dark cycles. The rhizobium strain Mesorhizobium loti MAFF 303099 was used for nodulation. Constructs and transformation p35S-CLE-RS1, p35S-CLE-RS2 and p35S-GUS constructs reported previously [16] were used to produce stably transformed plants that constitutively expressed either CLE-RS1 or CLE-RS2. For overexpressing LjIPT3 , the LjIPT3 open-reading frame fragment was amplified from MG-20 genomic DNA using the specific primer set (5′- CACCGATCAGATACCAATTTTGCA -3′ and 5′- ACCACCCTCTATGAACATAACTAAC -3′), and cloned into the pENTR/D-TOPO vector (Invitrogen). The insert was placed downstream of the p35S promoter of pH7WG2D [50] by LR clonase (Invitrogen). For promoter analysis of LjIPT3 , the 2-kb DNA fragment upstream of the putative translation initiation codon was cloned into the pENTR/D-TOPO vector and transferred to pGWB3 (ref. 51 ) by the Gateway LR reaction. The promoter fragment was amplified from MG-20 genomic DNA using the specific primer set (5′- CACCTTTGGTAATTGAATTTAATGGGCA -3′ and 5′- GGTGAATTGCAAAATTGGTATCTGATC -3′). Resultant binary vectors were introduced into Agrobacterium tumefaciens strain AGL1 and transformed into MG-20 as described previously [52] . Grafting experiments Seeds were sown on vertical 1% agar plates and grown for 2 days in darkness. Plants were further cultured for 2 days in 16 h light per 8 h dark cycles. Rootstocks were produced by cutting off the hypocotyl at its base. A short vertical slit (~2 mm) was made in the basal hypocotyl stump with a scalpel blade. A shoot scion was inserted into this vertical slit. Grafted plants were grown on filter papers saturated with sterilized water in Petri dishes for 4 days, before transfer to vermiculite supplemented with B&D solution and 0.5 mM KNO 3 (ref. 18 ). Quantification of phytohormones Shoots of 2-week-old plants (about 100 mg fresh weight) were collected 3 days after inoculation with M. loti , frozen in liquid N 2 and stored at −80 °C. Frozen shoots were crushed using a TissueLyser (Qiagen Retsch GmbH) with a zirconia bead (diameter, 5 mm) in a 2-ml microcentrifuge tube, and determination of primary metabolites was conducted according to Kojima et al . [53] In brief, the extract was passed through an Oasis HLB column (Waters), and the hormone-containing fraction was passed through an Oasis MCX column (Waters). Each of the phytohormones were eluted with methanol (elution 1), 0.35 M ammonia (elution 2) and 0.35 M ammonia in 60% (v/v) methanol (elution 3). The elution 1 fraction was passed through a DEAE-cellulose column (Vivapure D Mini M, Vivascience). Phytohormones were measured using a liquid chromatography-tandem mass chromatography system (ACQUITY UPLCSystem/Quattro Ultima Pt; Waters) with an ODS column (ACQUITY UPLC BEH C 18 , Waters). Determined phytohormones were trans -zeatin (tZ); tZ riboside (tZR); tZR 5′-phosphates (tZRPs); cis -zeatin (cZ); cZ riboside (cZR); cZR 5′-phosphates (cZRPs); dihydrozeatin (DZ); DZ riboside (DZR); DZ riboside 5′-phosphates (DZRPs); N 6 -(Δ 2 -isopentenyl) adenine (iP); iP riboside (iPR); iPR 5′-phosphates (iPRPs); tZ-7- N -glucoside (tZ7G); tZ-9- N -glucoside (tZ9G); tZ- O -glucoside (tZOG); cZ- O -glucoside (cZOG); tZR- O -glucoside (tZROG); cZR- O -glucoside (cZROG); tZRPs- O -glucoside (tZRPsOG); cZRPs- O -glucoside (cZRPsOG); DZ-9- N -glucoside (DZ9G); iP-7- N -glucoside (iP7G); iP-9- N -glucoside (iP9G); gibberellin (GA); salicylic acid (SA); jasmonic acid (JA); indole-3-acetic acid (IAA); abscisic acid (ABA). Quantification of CKs Shoots of 2-week-old plants (about 100 mg fresh weight) were collected 5 days after inoculation with M. loti (infection treatment) or application of B&D solution in the absence of rhizobia (non-infection treatment), frozen in liquid N 2 and stored at −80 °C. Frozen shoots were crushed using a TissueLyser with a zirconia bead in a 2-ml microcentrifuge tube, and determination of CK contents was conducted according to Kojima et al . [53] The CK quantification method was the same as the phytohormones quantification method described above. CK-feeding assay The distal half of a cotyledon was removed from 2-day-old seedlings grown on vermiculate. The remaining cotyledon stump was inserted into a plastic tube filled with 10 mM MES (pH 6.2) containing BAP. On the next day, plants were inoculated with rhizobia. The number of nodules was counted 2 weeks after inoculation. Expression analysis Total RNA was isolated from plants using the Concert Plant RNA Reagent (Invitrogen). First-strand complementary DNA was synthesized using the QuantiTect Reverse Transcription Kit (Qiagen). Real-time reverse transcriptase-PCR was performed on an ABI prism 7000 sequence detection system (Applied Biosystems) using the THUNDERBIRD SYBR qPCR Mix (Toyobo) according to the manufacturer’s protocol. The primers used are listed in Supplementary Table 3 . Expression of ubiquitin served as the reference. GUS assay Leaves were incubated in 90% acetone for 15 min at −20 °C, and then incubated with GUS-staining buffer (0.5 mg ml −1 X-gluc, 100 mM phosphate buffer) [54] for 24 h at 37 °C. The samples were washed twice with 100 mM NaPO 4 (pH 7.0), bleached with 70% ethanol at room temperature and dehydrated in 100% ethanol. Then the samples were embedded in Technovit 7100 resin (Haraeus Kulzer) according to the manufacturer’s protocol and sectioned (10 μm thickness) using a Microtome RM2255 (Leica). The sections were stained with 0.02% toluidine blue (Sigma) before observation. CK transport assay The distal half of each cotyledon was excised from seedlings grown for 3 days on 1% agar plates. Three μl of 0.5% agar containing 100 pmol isotope-labelled iPR, [ 13 C 10 , 15 N 5 ]N 6 -(Δ 2 -isopentyl) adenine riboside (Sakakibara laboratory, RIKEN Center for Sustainable Resource Science) [28] , were put on the cut surface of each cotyledon. Plants were placed vertically on sterilized filter paper saturated with sterilized water in Petri dishes for 4 h. Twenty root tips (2 mm) were collected and stored at −80 °C. Frozen root tips were crushed using a TissueLyser with a zirconia bead in a 2-ml microcentrifuge tube and CK contents were quantified as previously described [53] . The method was the same as the phytohormones quantification method described above. How to cite this article : Sasaki, T. et al . Shoot-derived cytokinins systemically regulate root nodulation. Nat. Commun. 5:4983 doi: 10.1038/ncomms5983 (2014). Accession codes: The nucleotide sequences reported in this paper have been submitted to the NCBI database with accession numbers: LjIPT1 , DQ436462; LjIPT2 , DQ436463; LjIPT3 , DQ436464; LjIPT4 , DQ436465; LjIPT5 , ABW77761; LjIPT9 , EEE85226.2.